Ecology ofEndozoicomonadaceaein three coral genera across the Pacific Ocean 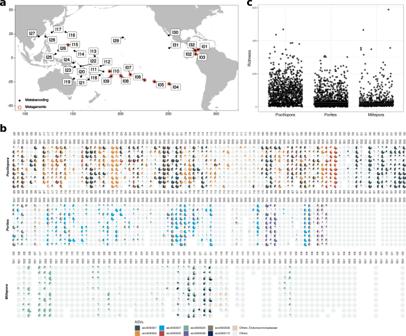Fig. 1:Endozoicomonadaceaedistribution and abundance in corals across the Pacific. aMap showing the islands sampled during theTaraPacific expedition. Black and red symbols indicate whether samples were analyzed by metabarcoding (16S rRNA gene) and/or metagenomics.bProportion of the most abundantEndozoicomonadaceaeASVs inPocillopora, Porites, andMilleporasampled across 99 reefs from 32 islands across the Pacific Ocean. The islands are ordered longitudinally from west to east.cEndozoicomonadaceaecommunity richness in the coralsPocillopora(n= 959 samples), Porites(n= 944), andMillepora(n= 544). The box plot horizontal bars show the median value, the box indicates the first and third QRs, and the whiskers indicate 1.5*IQR. Source data are provided as a Source Data file. Health and resilience of the coral holobiont depend on diverse bacterial communities often dominated by key marine symbionts of the Endozoicomonadaceae family. The factors controlling their distribution and their functional diversity remain, however, poorly known. Here, we study the ecology of Endozoicomonadaceae at an ocean basin-scale by sampling specimens from three coral genera ( Pocillopora , Porites , Millepora ) on 99 reefs from 32 islands across the Pacific Ocean. The analysis of 2447 metabarcoding and 270 metagenomic samples reveals that each coral genus harbored a distinct new species of Endozoicomonadaceae . These species are composed of nine lineages that have distinct biogeographic patterns. The most common one, found in Pocillopora , appears to be a globally distributed symbiont with distinct metabolic capabilities, including the synthesis of amino acids and vitamins not produced by the host. The other lineages are structured partly by the host genetic lineage in Pocillopora and mainly by the geographic location in Porites . Millepora is more rarely associated to Endozoicomonadaceae . Our results show that different coral genera exhibit distinct strategies of host- Endozoicomonadaceae associations that are defined at the bacteria lineage level. Tropical coral reefs are hotspots of biodiversity in the world’s oceans. They provide food and shelter for many marine animals, and are important to humans who benefit from the reefs’ goods and services [1] . In recent decades, global warming and human activities have, however, increasingly threatened coral reefs [2] , [3] , [4] , [5] . Their resilience and adaptability rely heavily on their ecosystem engineers, the corals, and their ability to resist damaging perturbations. In turn, the coral’s adaptive capabilities are anchored in its relationship with associated microorganisms that together with the host form the holobiont [6] , [7] , [8] , [9] . Coral holobionts include complex microbial communities composed of viruses, fungi, archaea, bacteria and micro-algae [10] . The symbiosis between the Symbiodiniaceae algae and corals is the best characterized association within the coral holobiont [11] , but bacteria are also important partners. Coral-associated bacteria contribute significantly to the health of the host by participating in nutrient acquisition, metabolic (re)cycling, and protection against pathogens [6] , [7] , [12] , [13] . Understanding the composition, the diversity and the functions of coral-associated microorganisms can thus provide clues about the health status, but also the resilience and adaptive capabilities of corals [14] . Among the large diversity of coral-associated bacteria [15] some are noteworthy because of their abundance and commonness. Bacteria from the Endozoicomonadaceae family ( Gammaproteobacteria, Oceanospirillales ) are frequent in corals [7] , [16] , but also in a number of other marine invertebrates such as sponges [17] , [18] , bivalves [19] , ascidians [20] or gorgonians [21] . Their global distribution in a large number of hosts make them potential key bacterial symbionts in the marine ecosystem [16] . An strict host-bacteria interdependency remains, however, to be demonstrated since Endozoicomonadaceae have some characteristics of non-obligate symbionts including possible free-living stages [22] , and relatively large genome sizes [23] , [24] . The family Endozoicomonadaceae was described only recently [25] and comprises the genera Parendozoicomonas [25] , Kistimonas [26] , Sansalvadorimonas [27] and Endozoicomonas [28] . Although the definition of the genus Endozoicomonas is recent, retrospective analysis show that it was commonly detected in early coral microbiome studies [29] , [30] , [31] , [32] , and it continues to be frequently reported in a number of different coral species [23] , [33] , [34] , [35] , [36] , [37] , [38] , [39] , [40] , [41] , [42] . Different corals may harbor different Endozoicomonadaceae 16S rRNA types that could show patterns of co-phylogeny with the coral host [41] , [43] . The patterns of host-symbiont associations have also been hypothesized to be linked to the reproductive mode of the host [43] , or the environmental condition [44] , while other studies suggest a correlation between Endozoicomonas and Symbiodiniaceae [45] . The question of host-specificity remains open, however, since some Endozoicomonadaceae types could be shared between different hosts [41] , different Endozoicomonadaceae types can dominate within a same host [43] , and changes in their relative abundance seems to be independent of the symbiotic algae [46] . If the host is not the driver of microbiome composition, external factors could play a role [47] . Endozoicomonadaceae communities could be shaped by environmental factors as they were shown to be less abundant in Acropora millepora at lower seawater pH [48] , [49] , or during increased temperatures and subsequent bleaching [31] , [50] , as well as anthropogenic impact and habitat suitability [44] , [51] . In Porites astreoides , lesioned colonies also contained fewer Endozoicomonas sequences, compared to non-lesioned colonies [52] . These findings suggest that Endozoicomonas are underrepresented in stressed corals [14] , however, it’s not always the case. In Pocillopora verrucosa and Acropora hemprichii , although Endozoicomonadaceae decreased at sites impacted by sedimentation, they increased at sites impacted by municipal wastewater [39] . Endozoicomonadaceae also increased in abundance in Porites spp. under lower pH [53] , and under natural stressful conditions of shallow hydrothermal vent [54] , and were not impacted by coral bleaching or severe tissue sloughing in P. verrucosa in response to eutrophication [55] . Endozoicomonadaceae also proliferated after warm summer months in French Polynesia [42] . These contrasted observations between individual studies conducted locally illustrate the need for a large-scale approach on multiple coral species to unveil Endozoicomonadaceae diversity and biogeography, and better understand the factors controlling their presence and community composition. The widespread prevalence of Endozoicomonadaceae in corals indicates that they are important for the host, and the analyses of their genomes have given some clues regarding their potential interactions and the establishment of symbiosis with corals [56] . Endozoicomonadaceae have large genome sizes that suggest a possibility for a non-symbiotic living stage before host invasion [23] , [24] , [57] . Host infection could be promoted by type III secretion system, like the one detected in a strain of Endozoicomonas montiporae [57] , and by potential effector proteins that that could help interactions [23] , [56] , [58] . A comparative analysis of several Endozoicomonadaceae genomes showed an enrichment of genes associated with carbon sugar transport and utilization, protein secretion, and synthesis of amino acids that could potentially be transferred to the host [43] . In addition, Endozoicomonas acroporae has the potential to degrade dimethylsulfoniopropionate (DMSP), which bacteria could use as a carbon source [24] . Various studies also suggested that Endozoicomonadaceae play a role in regulating the overall microbiome structure either by direct competition with other bacteria, or by producing antimicrobial compounds [48] , [59] . The extent of metabolic capabilities of Endozoicomonadaceae across species remains, however, to be mapped, and the variability of these pathways at ocean scale is not known. In this work, we study the ecology of Endozoicomonadaceae at an ocean-basin scale and in different coral genera. Our hypothesis was that different corals may have evolved different strategies of host-bacteria relationships. To assess this, we conducted an unprecedented campaign to methodically sample three globally distributed coral species. Based on morphology, we targeted the complex Pocillopora meandrina , the robust Porites lobata , and the fire coral Millepora platyphylla on 99 reefs from 32 islands across the Pacific Ocean. We precisely described the diversity of Endozoicomonadaceae in more than 2400 coral colonies by metabarcoding the 16S rRNA gene. In addition, we sequenced 270 metagenomes to assemble high-quality draft genomes of novel Endozoicomonadaceae species, and putative lineages. Here we show that the most common Endozoicomonadaceae lineage, found in Pocillopora , is globally distributed and has distinct metabolic capabilities, including the synthesis of amino acids and vitamins not produced by the host. The other lineages are structured partly by the host genetic lineage in Pocillopora and mainly by the geographic location in Porites . Our results demonstrate that different coral genera exhibit distinct strategies of host- Endozoicomonadaceae associations that are defined at the bacteria lineage level. Endozoicomonadaceae distribution and abundance in corals and seawater across the Pacific Ocean Overall, Endozoicomonadaceae ASVs were detected in 99% of the coral samples (n = 2447). Despite their prevalence, their relative abundance varied greatly between samples (Fig. 1b ). Pocillopora had the highest proportion of ASVs affiliated to Endozoicomonadaceae (53% of all Pocillopora sequences) followed by Porites (30%) and then Millepora (11%). Pocillopora also had the highest Endozoicomonadaceae richness, followed by Porites and then Millepora (Fig. 1c ). In Pocillopora , Endozoicomonadaceae were present in all islands, but with low relative abundances in Coïba (I02), Malpelo (I03), and Guam (I15). In Porites , Endozoicomonadaceae were not detected east of Rapa Nui (I04), and in Kiribati (I13) and Southwest Palau Islands (I25). In Millepora , Endozoicomonadaceae were almost absent in corals from islands located east of Fiji (I18), with the exception of Samoa (I10), and almost absent from Guam (I15) and Ogasawara Islands (I16). We observed high variations in relative abundance between sites in some islands, like in Las Perlas (I01), Cook (I08) and Kiribati (I13) for Pocillopora , and Gambier (I06), Upolu (I10) and Chuuk Island (I14) for Porites , and New Caledonia (I21), Southwest Palau Islands (I25) for Millepora . In other cases, there was a high relative abundance and low variability between sites (Fig. 1b ). At any given site, the presence of Endozoicomonadaceae in one coral genus was not predictive of its presence in the other genera (e.g., Rapa Nui I04 or Moorea I07), although at other sites, Endozoicomonadaceae were present and abundant in all three coral genera (e.g., Chesterfield I20 and New Caledonia I21). Fig. 1: Endozoicomonadaceae distribution and abundance in corals across the Pacific. a Map showing the islands sampled during the Tara Pacific expedition. Black and red symbols indicate whether samples were analyzed by metabarcoding (16S rRNA gene) and/or metagenomics. b Proportion of the most abundant Endozoicomonadaceae ASVs in Pocillopora, Porites , and Millepora sampled across 99 reefs from 32 islands across the Pacific Ocean. The islands are ordered longitudinally from west to east. c Endozoicomonadaceae community richness in the corals Pocillopora ( n = 959 samples) , Porites ( n = 944), and Millepora ( n = 544). The box plot horizontal bars show the median value, the box indicates the first and third QRs, and the whiskers indicate 1.5*IQR. Source data are provided as a Source Data file. Full size image Overall, asv0000001 was the most abundant Endozoicomonadaceae (12% of the sequences in the dataset) and the most common (found in 78% of the samples) (Fig. 2 ). Pocillopora had 3 dominant ASVs (abundance >1%, asv0000001, asv0000003, asv0000020) of which asv0000020 was more abundant at Rapa Nui (I04) and asv0000003 at the Great Barrier Reef (I19) (Fig. 1 ). Porites also had 3 dominant ASVs (asv0000007, asv0000028, asv0000038); asv0000028 dominated at Ducie Island (I05) and Niue (I09). Millepora had two dominant ASVs (asv0000024, asv0000110), of which asv0000110 was found mostly in Chesterfield (I20), New Caledonia (I21) and Solomon Islands (I22)(Fig. 1 ). All dominant ASVs had a broad geographic distribution since the same ASVs were found across the entire Pacific Ocean. Each of the ASVs defined as dominant in one coral host were also detected at very low proportions (>0.1%) in the other coral species (Fig. 2 ). Fig. 2: Prevalence and relative abundance of Endozoicomonadaceae. Endozoicomonadaceae ASVs found in a all corals, b Pocillopora, c Porites and d Millepora. Full size image When the relative abundance of Endozoicomonadaceae in corals was low, the diversity of the overall microbial community reached higher values (Supplementary Fig. 1a ). In Pocillopora , corals with low abundance of Endozoicomonadaceae were often dominated by Flavobacteriaceae (Supplementary Fig. 1b ). In Porites , there were more Kiloniellaceae and Rhodobacteraceae , while in Millepora there were more Spirochaetaceae . We also looked for Endozoicomonadaceae ASVs in the water surrounding the Pocillopora colonies, in surface water over the reef, and in the surface water off the island (Fig. 3 ). Endozoicomonadaceae sequences were detected in the water, but their relative abundance decreased rapidly with increasing distance from the colonies (Fig. 3a ). While Endozoicomonadaceae represented on average 30% of the bacteria in Pocillopora , their relative abundances decreased to ~0.5% in coral surrounding water, 0.05% in surface water over the reef, and 0.001% in surface water off the island (Fig. 3a ). Additionally, we observed a significant positive correlation ( r = 0.52) between the relative abundance of Endozoicomonadaceae in Pocillopora and in the colony surrounding water (Fig. 3b ). The Endozoicomonadaceae ASVs that were abundant in Pocillopora were also detected in the water, but in varying proportions (Fig. 3c ). When moving away from the Pocillopora colonies, the proportion of typical Pocillopora Endozoicomonadaceae (asv0000001, asv0000003 and asv0000020) decreased, while the proportion of other Endozoicomonadaceae increased. In some cases, Endozoicomonadaceae were not detected at all in the surface water off the island. Fig. 3: Relative abundance of Endozoicomonadaceae in Pocillopora corals and the surrounding environment. a Endozoicomonadaceae relative abundance in the coral Pocillopora host, the colony surrounding water (CSW), the surface water over the reef (rSRF), and the surface water off the island (iSRF) in the 0.2–3 µm planktonic size fraction. The box plot horizontal bars show the median value, the box indicates the first and third QRs, and the whiskers indicate 1.5*IQR. b Spearman correlation between relative abundance of Endozoicomonadaceae in Pocillopora and in colony surrounding water (CSW). The lines represent the result of linear regression with the gray shadow as the 95% confidence interval. A two-sided p -value is given. c Relative abundance of the dominant Endozoicomonadaceae ASVs in the different sampling environments at each island. Source data are provided as a Source Data file. Full size image Correlation between Endozoicomonadaceae , environment, islands, host genetic lineages, Symbiodiniaceae symbionts, and phylotypic biomarkers There was no strong correlation between Endozoicomonadaceae relative abundance at the family level and chlorophyll a, pH, phosphate, silanol, sea surface salinity and temperature in Pocillopora and Millepora (Fig. 4a ). In Porites, Endozoicomonadaceae had the highest correlation to salinity. At the ASV level, however, all correlation values were low, but there were differences within coral genera. In Pocillopora , asv0000001 had the strongest positive correlation to sea surface temperature and was negatively associated with pH, while asv0000003 and asv0000020 had the highest correlations to salinity and were negatively correlated to SiOH (Fig. 4a ). In Porites , asv0000007 had the highest positive correlation to salinity, while asv0000028 and asv0000038 only had very low correlation values to environmental conditions. In Millepora , asv0000024 had the highest positive correlation to SiOH and asv0000110 only had low correlation values (Fig. 4a ). Fig. 4: Correlation between Endozoicomonadaceae , environment, islands, host genetic lineages, Symbiodiniaceae symbionts, and phylotypic biomarkers. a Kendall correlations across 32 islands between abundant Endozoicomonadaceae ASVs and environmental factors. Pocillopora ( n = 889 samples), Porites ( n = 903), and Millepora ( n = 515). SST: Sea Surface Temperature; SiOH: Silanol; chl: Chlorophyll a; SSS: Sea Surface Salinity; pH; PO4: phosphate. b Mantel correlation across 11 islands between Endozoicomonadacea community composition and environmental conditions, phylotypic biomarkers, Symbiodiniaceae assemblages and coral host genetic lineages for the two coral genera Pocillopora ( n = 77) and Porites ( n = 80) phylotypic biomarkers data for Millepora are missing). c Variance partition analysis explaining the variance of the relative abundance of Endozoicomonadaceae and individual ASVs across 11 islands in relation to island, coral genetic lineages and Symbiodiniaceae assemblages in Pocillopora ( n = 96) , Porites ( n = 99),and Millepora ( n = 55). Source data are provided as a Source Data file. Full size image Information about assemblages of Symbiodiniaceae, phylotypic biomarkers indicative of coral health, and host genetic lineages was obtained from a subset of 11 islands (Fig. 1a —red circle). The host genetic lineages identified through genome-wide SNP calling (material and methods) separated Pocillopora in five genetic lineages (Poc-SVD1 to Poc-SVD5), Porites in nine lineages (Por-K1a to Por-K3d) and Millepora in six lineages (Mil-SVD1 to Mil-SVD6). Overall, the composition of Endozoicomonadaceae communities was best explained by the genetic lineage of the host for both Pocillopora and Porites (Fig. 4b ). Symbiodiniaceae had low significance with regard to Endozoicomonadaceae assemblage in Pocillopora , and the environment had low significance in Porites . Phylotypic biomarkers were always the lowest explanatory factor. At the ASV level, variance partitioning showed that individual ASVs had a higher proportion of variance explained than overall Endozoicomonadaceae (Fig. 4c ). For Pocillopora , asv0000001 and asv0000003 had the largest proportion of their variation explained by the factor ‘island’, while asv0000020 was explained mostly by the genetic lineage of the host (Fig. 4c ). In Porites , the overall Endozoicomonadaceae relative abundance was best explained by the host genetic lineage, but all individual ASVs (asv0000007, asv0000028 and asv0000038) had most of their variance explained by island. Asv0000038 had only a small portion of the variance explained by the factors that we tested. In Millepora , the Symbiodiniaceae assemblage was the strongest explanatory factor for both asv0000024 and asv0000110. On the 11 islands we could also correlate individual ASV relative abundance to individual coral biomarkers. Different ASVs showed distinct correlation patterns (Supplementary Fig. 2 ). In Pocillopora , asv0000001 had strongest positive correlations to Symbiodiniaceae cell content and negatively to protein carbonylation (Supplementary Fig. 2 ). Asv000003 was positively correlated to total antioxidant content and asv0000020 to protein ubiquitination. In Porites , asv0000007 was most positively correlated to Symbiodiniaceae content, and asv0000038 to protein carbonylation (Supplementary Fig. 2 ). Genomic characteristics and phylogeny of Endozoicomonadaceae A total of 270 coral metagenomes were sequenced from a subset of 11 islands covering 33 reefs (Fig. 1 a). We reconstructed a total of 24 MAGs belonging to the Endozoicomonadaceae family. They had a completeness ranging from 51.2% to 93.3%, and contamination levels from 0% to 4.9% (Supplementary Data 1 ). To conduct comparative genomics analyses, all publicly available Endozoicomonadaceae genomes were downloaded from NCBI or recovered from the literature ( n = 30). The taxonomic annotation of the MAGs and the phylogenetic tree based on 71 marker genes separated the Endozoicomonadaceae into five distinct genera: Endozoicomonas, Parendozoicomonas, Kistimonas, Sansalvadorimonas , and one unnamed genus (Fig. 5 , Supplementary Data 1 ). Our Tara Pacific MAGs fell within two of these genera: the Endozoicomonas genus for Millepora and Pocillopora MAGs, and the Parendozoicomonas genus for Porites MAGs. All Endozoicomonadaceae genomes had similar coding density (80.8–91.6%), but distinct guanine-cytosine (GC) contents (33.2–57.3%) between genera (Supplementary Data 1 ). Endozoicomonas and Parendozoicomonas had similar GC contents with, respectively, 48.5% and 48.2%, while the only Kistimonas and Sansalvadorimonas genomes available had 57.3% and 50.3%, respectively (Supplementary Data 1 ). Fig. 5: Distance tree of Endozoicomonadaceae. a Based on 71 concatenated single-copy marker proteins from MAGs and b based on 16S rRNA genes from ASVs. Clades were defined in this study. ASVs and MAGs from this study are in bold. c Proportion of ASVs in the samples from which the MAGs were reconstructed. Full size image The Parendozoicomonas genomes formed a monophyletic group with average ANI and AAI values of 73.80% (73.41–74.12%) and 71% (70.33–71.41%), respectively (Supplementary Fig. 3 , Supplementary Data 2 ). The Endozoicomonas genomes also formed a well defined group, and they had average ANI and AAI values of 76% (71.08–99.99%) and 73% (60.96–99.99%), respectively. The genus Sansalvadorimonas has only one representative, Sansalvadorimonas verongulae . Because its genome is not present in the latest version of GTDB database, it was first annotated as Parendozoicomonas , but our genomic analysis confirmed its position as a distinct genus. Our Tara Pacific MAGs from Pocillopora , Porites , and Millepora were divided into three well-supported monophyletic clusters that corresponded to the three coral hosts (Fig. 5a , Supplementary Fig. 3 ). Endozoicomonas MAGs obtained from Pocillopora all grouped with sequences from the Pocilloporidae family earlier obtained from one P. verrucosa and two S. pistillata [23] . The two Endozoicomonas genomes from S. pistillata represent two distinct species (93% ANI similarity). Parendozoicomonas MAGs from Porites clustered with a MAG obtained earlier from Porites lutea [12] . It was previously annotated as Endozoicomonas , but our analysis shows that it is a Parendozoicomonas with closer similarity to Parendozoicomonas from P. haliclonae (73.8% ANI and 70.69% AAI) than with other Endozoicomonas genomes (71.83% ANI and 60.50% AAI). Millepora MAGs were distantly related to all genomes published to date (Fig. 5a ). Although Endozoicomonas genomes from the same host species clustered together, there was no clear pattern of co-phylogeny between the bacteria and their host . Endozoicomonas genomes from different coral genera were often more related to genomes from other marine invertebrates (Supplementary Fig. 3 ). For instance, the Endozoicomonas symbionts of two Acropora species , A. humilis and A. muricata , were separated in two distinct clades and were more closely related to a sponge and an ascidian symbiont than to each other. There were, however, exceptions and Endozoicomonas symbionts from S. pistillata, P. verrucosa , and P. meandrina clustered according to host phylogeny. In the MAGs from this study, ANI was >95% in coral host-specific clusters, which corresponds to the threshold used for species delineation [60] . The specI method confirmed that each coral species harbored one specific Endozoicomonadaceae species (Supplementary Data 1 ). We could also delineate subclades within host-specific Endozoicomonadaceae species. Within Pocillopora , the MAGs were separated into three subclades that corresponded to three distinct Pocillopora genetic lineages (Poc-SVD5, Poc-SVD1 and Poc-SVD3) (Fig. 5c ). For Porites , the MAGs separated into 6 subclades (Fig. 5c ). The subclades that contained most MAGs corresponded exclusively to the Porites genetic lineages K3b. For Millepora , all MAGs shared a high identity and thus belonged to the same group. Based on the phylogenomic tree, SpecI results and ANI/AAI values we thus propose three new species of Endozoicomonadaceae : Candidatus Endozoicomonas pocilloporae sp. nov., Candidatus Parendozoicomonas poriteae sp. nov and Candidatus Endozoicomonas milleporae sp. nov. Additionally, we propose three lineages within E. pocilloporae , Poc - SVD1, Poc-SVD3 and Poc - SVD5, named according to the host genetic lineages (Fig. 5c , Supplementary Fig. 4 ). We also propose 6 lineages within P. poriteae , also named according to lineages, of which Por-K3c2 was not host lineage specific (Fig. 5c ). We constructed a phylogenetic tree based on 16S rRNA gene sequences (ASVs) obtained from Tara Pacific amplicon sequencing data and references from the literature. The 16S rRNA gene tree had a similar topology than the marker gene tree (Fig. 5b ) separating the 4 named Endozoicomonadaceae genera. ASVs from the 3 coral species were separated in host-specific clades under the Endozoicomonas and Parendozoicomonas genera. Within host-specific clades, ASVs grouped in distinct subclades. For Pocillopora , we delineated 3 clades. Clade A included the most common ASV (asv0000001), as well as sequences from Pocillopora of the Red Sea (clone P4-B01, KC668593 [36] ). Clade A was found in most Pocillopora genetic lineages (Supplementary Fig. 5 ). Clade B contained asv0000020 found mostly in the genetic lineage SVD5. Clade C contained asv0000003, as well as sequences from the Great Barrier reef (clone PDA-OTU2, AY700600 [30] ) (Fig. 5b ), and was found mostly in host lineages SVD1, SVD2 and SVD5 (Supplementary Fig. 5 ). For Porites , we delineated 3 groups. The most common ASV was in clade D (asv0000007) together with a sequence from the Indian Ocean (clone RSAE6C40, KF180129 [61] ); it was more common in genetic lineage K2. Other common ASVs were in clade E (asv0000028), clade F (asv0000038) that were more common in the Porites lineage K3 (Supplementary Fig. 5 ). Millepora ASVs grouped in two clades, clade G and H, corresponding to the two most common ASVs (asv0000024 and asv0000110) (Fig. 4b ). Since the Endozoicomonadaceae MAGs did not contain 16S rRNA genes, we could not directly link the genomes to the ASVs. However, by looking at the ASV relative abundance in the samples from which the MAGs were reconstructed, we could associate groups of ASVs to the MAGs (Fig. 5c ). In Pocillopora , the Endozoicomonas strains Poc-SVD1 and Poc-SVD3 corresponded to the dominance of asv0000001 (clade A), and Poc-SVD5 contained a majority of asv0000020 (clade B), but also asv0000003 (clade C). In Porites , Por-K3b, Por-K3c2 and Por-K3d had a majority of asv0000028 (clade E), while Por-K2b, Por-K2c and Por-K3c had more asv0000007 (D) (Fig. 5c ). Endozoicomonadaceae mOTUs and mTAGs Endozoicomonadaceae MAGs were also grouped into marker genes-based operational taxonomic units (mOTUs). All Parendozoicomonas MAGs from Porites grouped within one mOTU (mOTU_3), Endozoicomonas MAGs from Pocillopora were separated in two mOTUs (mOTU_2 and mOTU_67) and Millepora MAGs in one mOTU (mOTU_23) (Supplementary Fig. 6 ). Only one Endozoicomonas MAGs belonged to the mOTU_67 and was recovered from a SVD5 lineage coral while five of them grouped into the mOTU_2 and were recovered from SVD1 and SVD3 lineage corals (Supplementary Fig. 5 ). Finally, two MAGs did not have enough marker genes (<6) to be grouped into mOTUs. The mOTUs were specific to the coral host. The relative abundance of Endozoicomonadaceae were determined based on mOTUs and mTAGs, which are 16S rRNA gene sequences extracted from metagenomes, in our three different coral species from 11 islands across the Pacific Ocean (Supplementary Fig. 7 ). We observed broadly similar patterns between mOTUs, mTAGs and ASVs profiles. We detected, however, some small differences: mTAGs and ASVs allowed the detection of Endozoicomonadaceae at very low abundance that were not seen with mOTU in Coiba (I02) and Guam (I15) islands for Pocillopora , in Coiba (I02), Cook (I08) and Rapa Nui (I04) for Porites and in Moorea (I07), Cook (I08), Niue (I09) and Guam (I15) islands for Millepora (Fig. 1 , Supplementary Fig. 7 ). Metabolic capabilities of Endozoicomonadaceae Among the pathways common to all Endozoicomonadaceae we noted the Embden-Meyerhof pathway, the pyruvate dehydrogenase, the citrate cycle, the non-oxidative phase of the pentose phosphate pathway, and the Type I, II secretion systems. Sequences coding for subunits of the DmsABC enzyme, which catalyzes the reduction of dimethylsulfoxide (DMSO) to dimethyl sulfide (DMS), were also detected in all Endozoicomonadaceae (Fig. 6 , Supplementary Fig. 8 ). Most Endozoicomonadaceae encoded different eukaryotic-like proteins (ankyrin, leucine-rich, tetratricopeptide, HEAT and WD40 repeats). We did not find any genes involved in the assimilation of nitrate in the E. pocilloporae, P. poriteae , and E. milleporae , species, but they were present in E. acroporae and P. haliclonae (Supplementary Fig. 8 ). Fig. 6: Schematic summary of the inferred metabolisms and appendages characterizing the three new species and lineages (SVD5, K3c1) of Endozoicomonadaceae found in Pocillopora (orange), Porites (blue), and Millepora (green) . Underlined names: vitamin or amino acid also produced by the coral host, asterisk: genes for export not known. T6SS: type 6 secretion system, ELP: eukaryotic like protein, ARPs: actin-related proteins, LRR: leucine-rich repeats, DMSP: dimethylsulfoniopropionate, DMSO: dimethylsulfoxide, DMS: Dimethyl sulfide. Full size image The three new Endozoicomonadaceae genomes had genes for biotin (vitamin B7) biosynthesis, from pimeloyl-Coa and the pimeloyl-[acp], and export (Supplementary Fig. 9a ). The biosynthesis pathway of the pimeloyl precursor through the BioI, BioW and BioC-BioH pathways were, however, incomplete in all the Endozoicomonadaceae genomes. The genes to synthesize this precursor through BioI (long chain acyl pathway) were present in all the genomes of the coral hosts that we analyzed (Supplementary Fig. 9b ). Most of the Endozoicomonadaceae genomes had genes for the biosynthesis of riboflavin (vitamin B2). E. milleporae and P. poriteae had the potential to export riboflavin, but not E. pocilloporae (Supplementary Fig. 9 , Fig. 6 ). Genes for the synthesis of the two flavoproteins, derived from riboflavin, the flavin adenine dinucleotide (FAD) and the flavin mononucleotide (FMN) were found in all three Endozoicomonadaceae (Supplementary Fig. 9 ). The genes for riboflavin synthesis were not present in our coral host genomes (Supplementary Fig. 9b ). E. pocilloporae and P. poriteae also had the potential to synthesize thiamine (vitamin B1), while the coral host could not. Finally, E. pocilloporae and E. milleporae and the coral hosts had the potential of folate (vitamine B9) synthesis (Supplementary Fig. 9b ). Alanine and phenylalanine biosynthesis, and their potential export by genes with an AlaE and EamA domain, were found in the three Endozoicomonadaceae species (Fig. 6 , Supplementary Fig. 10 ). Only E. pocilloporae and P. poriteae harbored genes for the cysteine synthesis, and had the potential to export it through the cydDC complex or bcr gene. Only E. pocilloporae and E. milleporae had genes involved in the biosynthesis of methionine as well as genes with AzlCD domains, which could allow the export of the amino acid. Genes for serine (Ser) biosynthesis were present in P. poriteae and E. pocilloporae Poc-SVD5 and Poc-SVD3. Threonine (Thr) biosynthesis were present in some P. poriteae and E. pocilloporae . However, genes for export with ThrE domains (Thr and Ser export) were only found in P. poriteae . Tryptophan (Trp) biosynthesis genes were found only in P. poriteae that also had the gene carrying the EamA domain for putative Trp export. The coral hosts only had the potential for alanine synthesis (Supplementary Fig. 10b ). Regarding motility, the presence of genes coding for pili and flagella varied between Endozoicomonadaceae. E. milleporae and P. poriteae did not have sequences for the flagella genes, while E. pocilloporae did . E. milleporae and P. poriteae had genes for the type IVb pilus, but E. pocilloporae did not. All had genes for the type IV pilus (Fig. 6 ). Some Endozoicomonadaceae , like E. montiporae and P. haliclonae , had all the genes for these three appendages (Supplementary Fig. 8 ). Type VI secretion system (T6SS) was only found in E. pocilloporae (Fig. 6 ). Among genes coding for transporters, phosphate, zinc and methionine transporters were found in the Endozoicomonadaceae genomes from the 3 coral species (Supplementary Fig. 8 ). Inversely, sequence coding for the transport of Arginine were found only in P. poriteae , and L-Amino acid transport genes only in E. pocilloporae (Supplementary Fig. 8 ). Genes for different subunits of the phosphotransferase system (PTS) were present in Endozoicomonadaceae . Most of the Endozoicomonadaceae species had the potential to assimilate fructose, glucose and beta-glucoside. Alpha-glucoside, trehalose and maltose PTS genes were found in E. pocilloporae and P. poriteae (Supplementary Fig. 8 ). E. pocilloporae and the Por-K3c1 clade of P. poriteae could assimilate cellobiose, while maltose assimilation potential was only present in the Poc-SVD5 clade within E. pocilloporae . Protein coding sequences for the degradation of chitin residue were detected in E. milleporae , E. pocilloporae and P. poriteae species. However, among chitin residues, E. milleporae has only the potential to assimilate a N-Acetylglucosamine (GlcNac) monomer, while E. pocilloporae and P. poriteae have the capabilities to assimilate GlcNac dimers (chitobiose) and trimers (chitotriose) (Supplementary Fig. 8 ). 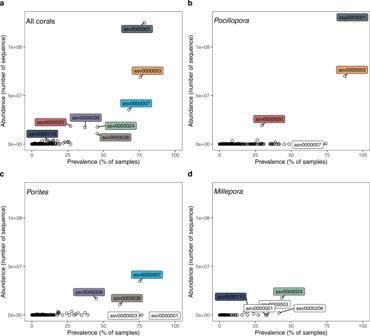Fig. 2: Prevalence and relative abundance of Endozoicomonadaceae. Endozoicomonadaceae ASVs found inaall corals,bPocillopora,cPorites anddMillepora. Although E. pocillporae and P. poriteae have the capability to actively import chitin oligomers (trimmer to hexamer) into their periplasm, only E. pocilloporae Poc-SVD5 has the chitinase gene to degrade GlcNac tretramer (Chitodextrine) and larger polymers. Among amino sugar metabolisms, N-Acetylmuramic acid (MurNac) phosphotransferase system was only detected in E. milleporae MAGs. MurNAc and GlcNAc can be both used for the biosynthesis of peptidoglycan, however, GlcNAc contrary to MurNAc can be redirected to the glycolysis pathway. Genes involved in the uptake of the L-Ascorbate (vitamin C) and its anaerobic degradation in D-Xylulose-5P were found in E. milleporae and P. poriteae only (Supplementary Fig. 8 ). The type II L-ascorbate degradation (aerobic) was partially complete. In fact only the genes common to anaerobic degradation were present. Key genes required for degrading testosterone were not detected in the E. milleporae , E. pocilloporae, and P. poriteae species. The Endozoicomonadaceae E. montiporae and E. elysicola had all genes required for the degradation of androstenedione, but E. pocilloporae , E. milleporae , and E. milleporae did not (Supplementary Fig. 8 ). E. milleporae , P. poriteae , and E. pocilloporae like E. elysicola genomes showed the potential for arsenate detoxification through the Type III arsenate detoxification and the arsenite methylation pathways (Supplementary Fig. 8 ). Almost all Endozoicomonadaceae species had the capabilities of heme B biosynthesis from the L-glutamate (Supplementary Fig. 8 ). However, for E. milleporae , the first protein involved in the pathway, which catalyzes the reaction of transforming L-Glutamate in L-Glutamate-tRNA was not found. Additionally, none of our recovered MAGs contains the genes allowing siroheme biosynthesis. The genes implied in heme A biosynthesis from the heme were found in all Endozoicomonadaceae species except for E. milleporae . The biosynthesis of biliverdin, another product of the heme, was found in most of the Endozoicomonadaceae species apart from E. milleporae , Kistimonas and genomes from the unnamed Endozoicomonadaceae genus (Supplementary Fig. 8 ). We also annotated the MAGs against the CAZy database specificaly targeting carbohydrate active enzymes. A PCA based on CAZy composition separated the Porites MAGs from Millepora and Pocillopora , which could not be separated from each other (Supplementary Fig. 11 ). The CAZy that best explained the separation between groups are listed in Supplementary Data 2 . The unprecedented systematic sampling effort of the Tara Pacific expedition revealed that each studied coral genus was closely associated with one specific Endozoicomonadaceae species with broad cross-ocean geographic distribution despite varying environmental conditions. These new host-specific bacteria were composed of different lineages that varied in proportion between reefs, and the lineages’ biogeography showed that the host-bacteria association patterns differed between host species. Endozoicomonadaceae strains had specific metabolic potentials, and they were associated with the host’s genetic lineage, or the islands, rather than to environmental conditions. Pocillopora Pocillopora was the coral genus that contained the highest proportion of Endozoicomonadaceae , and more precisely, it was specifically associated with the newly described species E. pocilloporae within the genus Endozoicomonas ( Supplementary discussion ). Among the three main E. pocilloporae strains, the most common, clade A (asv0000001, 90% of the Pocillopora samples), appears like an extremely successful coral-associated bacterium. It was abundant across the entire Pacific Ocean, and also found, although at very low relative abundance, in Porites and Millepora (in 82% of all coral samples), suggesting an important function in the coral holobiont (explored further below). The clade A sequence was similar to sequences found earlier in P. verrucosa and P. damicornis in the Red Sea and American Samoa [36] , [43] indicating the presence of a global E. pocilloporae strain shared between different Pocillopora species. We also identified sequences 100% identical to our clade A in earlier studies on the effect of stress on coral microbiomes. Our clade A corresponded to an abundant Pocillopora OTU that did not decrease in abundance under elevated nitrate and urea concentrations in the Pacific Ocean (Moorea) or the Red Sea [42] , [55] , although it decreased under excess dissolved organic carbon (OTU2 [55] ) and elevated temperature (OTU-Endo [62] ). The success of E. pocilloporae clade A may thus, in part, rely on its tolerance to specific environmental perturbations, but it could also benefit from its ability to disperse and effectively colonize corals. We found it abundant in the plankton surrounding the coral colonies, or ‘coral ecosphere’ [22] , and as far away as in water off the islands, yet in lower abundances. In addition, the genomes of E. pocilloporae harbour flagellar assembly genes, which are not found in P. poriteae and E. milleporae . The potential ability to produce a flagellum could allow bacteria to swim towards hosts [63] , [64] , and facilitate effective colonization of corals able to spawn like Pocillopora , which can acquire prokaryotes from the environment [56] , [65] , [66] , [67] , [68] . Finall y, E. pocillopor ae was also characterized by the presence of a type VI secretion system, an antibacterial apparatus delivering toxins [69] , that would give a competitive benefit by preventing other bacteria from multiplying in the coral host [70] . Clade A was, however, not always dominant. It was thought that Pocillopora was always associated with a single Endozoicomonas [43] , but our study reveals that other clades (16S rRNA gene clade B and C) replaced the dominant clade A in some islands. These clades were associated with specific genetic lineages of Pocillopora . Clade B (asv0000020) was most abundant in the genetic lineage SVD5 found in Easter Island (I04), where Clade A was completely absent. Clade B could represent a bacterium that has co-evolved with its SVD5 host. SVD5 was also present in Moorea (I07), but there, clade B was present in association with Clade A. The host-bacteria association could thus reflect an interplay between co-evolution that is strongly marked in isolated islands, such as Easter Island, and other selection factors leading to mixed communities, potentially via ‘shuffling’ of abundant Endozoicomonas phylotypes [71] in more interconnected islands. Clade C (asv0000003) was most abundant at the Great Barrier Reef (I19), and was closely related to a bacterium earlier detected in P. damicornis in eastern Australia [30] . Our field observations indicate that the corals sampled at the Great Barrier Reef during the Tara Pacific expedition may have been P. damicornis . Clade C could thus be specific to that coral species. Clade B and C had, together with clade A, the potential for type IV pili synthesis, which could help host sensing and surface motility [72] . Our genome analysis showed that E. pocilloporae have genes coding for the production of the essential vitamins B1, B2 and B7, and specific amino acids (Phe, Cys, Met), while the coral hosts did not have these metabolic capabilities. The coral holobiont must thus acquire these essential metabolites from heterotrophic feeding and/or its associated prokaryotes, including E. pocilloporae . Many algae like Symbiodiniaceae are auxotrophs for different B vitamins [12] , [56] , [73] , [74] and could also need vitamins produced by bacteria. Our data also provide clues about E. pocilloporae lifestyle. They had the genomic potential for cellobiose assimilation, suggesting that they could use cellulose originating from the degradation of Symbiodiniaceae cells [23] . However, our study also revealed differences in potential metabolisms between E. pocilloporae lineages. Poc-SVD1, contrary to Poc-SVD5 and Poc-SVD3, had the potential to degrade chitin, the most abundant polysaccharide in the ocean [75] , and which for instance could originate from zooplankton taken by the coral via heterotrophic feeding. The Poc-SVD5 genomes, corresponding to 16S rRNA gene Clade B and C defined in this study, had the potential to assimilate maltose, a sugar resulting from the hydrolysis of starch. Starch could originate from Symbiodiniaceae’s carbon and energy storage. Differences in maltose metabolisms between different E. pocilloporae lineages may thus reflect the presence of different Symbiodiniaceae genera that have different energy storage strategies, and thus different starch content [76] . Poc-SVD5 was associated with Symbiodiniaceae Cladocopium C42, while Poc-SVD1 was reconstructed from samples with higher proportion of Cladocopium C1. Porites In Porites , although Endozoicomonas was the most common and abundant bacterial symbiont, it was rare or absent from a large number of islands. Endozoicomonas has earlier been shown to be abundant in Porites from the Caribbean [34] , [38] and the Pacific Ocean [53] , but our data reveal that their overall abundance can vary greatly geographically. The pattern of host-bacteria association thus appears different from the one seen in Pocillopora , with different species of associated Endozoicomonadaceae . The new species P. poriteae , genus Parendozoicomonas , was dominated by Clade D (asv0000007) found from the Gambier Island (I06) to Sesoko Island in the west Pacific (I19). Clade D sequences were similar to the ones found earlier in the Indian Ocean off South Africa [61] indicating that its geographic spread is probably large. This wide geographic distribution, although not as extensive as E. pocillopora e Clade A, may also be due to resistance to some environmental perturbations. Sequence comparison showed that Endozoicomonas similar to clade D resisted elevated environmental nitrate and urea concentrations, and elevated temperatures [42] . In P. lobata , Endozoicomonadaceae , although we could not verify lineage identity, did not decline under nutrient stress [77] or elevated pH at CO 2 seeps [48] , [53] . Other P. poriteae lineages were more limited in their distribution, and contrary to E. pocilloporae , the distribution of these less abundant lineages was associated with islands rather than their host’s genetic lineage. Clade F was for instance mostly restricted to Ducie Island (I05) and Cook Island (I09). The P. poriteae genomes also showed differences to E. pocilloporae ; they had genes coding for a type IVb pilus for host colonization and adhesion [78] , and may be able to provide their host with B1, B2 and B7 vitamins, and Thr/Trp amino acids. Interestingly, there were also differences among the different P. poriteae lineages. Por-K3c1, which corresponded to asv0000007, was the only P. poriteae that had the potential for cellobiose assimilation. The Por-K3c1 lineage was also the only one to have a gene coding for metabolizing dimethylsulfoniopropionate (DMSP) into dimethyl sulfide (DMS). That gene was not found in other P. poriteae , E. pocilloporae or E. milleporae lineages, which indicates that the involvement of Endozoicomonadaceae in the sulfur cycle [24] is very much lineage specific. Millepora In Millepora , host-bacteria association differed from that of scleractinian corals, with only few sampled fire coral colonies having abundant communities of Endozoicomonas . The association seems looser and thus probably less important for the host. Among the 2 main E. milleporae lineages, clade G had the widest distribution, while clade H was more common in areas around New Caledonia (I21). Our analyses suggest that E. milleporae clades were associated with specific Symbiodiniaceae genera and coral host genetic lineages, but these results remain hypothetical since only few Endozoicomonas were present in the 11 islands for which host genetic information was available. Our results contrast with the ones from a recent study in Moorea [47] where differences in bacterial abundance were associated with reef habitats rather than host genotype. Similarly, in the soft coral Scleronephthya gracillium, Endozoicomonas abundance varied greatly along the Kuroshio Current Region, and was seemingly related to differences in reef habitats [79] . In our study, the environmental parameters did not strongly explain the variability of Endozoicomonas in Millepora . Regarding potential metabolisms, E. milleporae , contrary to E. pocilloporae and P. poriteae , did not have the potential to use GlcNac polymer, cellobiose or starch, but could use peptidoglycans from other bacteria. Our results draw a fine picture of the patterns of Endozoicomonadaceae abundance in corals across the Pacific Ocean with implications for our understanding of the ecology and evolution of host-symbiont relationships. We show that the ecology of this widespread symbiont should be considered at the lineage level to understand the factors structuring communities and infer associated metabolic contributions. Our data suggest that different coral species exhibit distinct host- Endozoicomonadaceae relationships ranging from a strong association illustrated by the global, and abundant presence of Endozoicomonas in Pocillopora , to a rather weak association with a rare and scattered presence in Millepora . In all corals, the environment had generally only a small structuring effect on Endozoicomonadaceae community composition, while the genetic lineage of the host was important in some corals, arguing for a high level of host specificity putatively shaped by long co-evolutionary histories. Thus, coral-bacterial association at large may range from stable co-dependent relationships that arose through evolutionary time to opportunistic associations that are flexible and determined by the prevailing environment. Even for bacteria within the family Endozoicomonadaceae , we find evidence for one and the other. Pocillopora was associated with a very abundant Endozoicomonas lineage throughout its entire geographic range. The success of this lineage could be explained by its functional potential inferred from genome characteristics including the ability to swim, destroy other bacteria, and thrive on carbon sources produced by Symbiodiniaceae. Other E. pocilloporae lineages were specific to the host’s genetic lineages, while in P. poriteae , the lineages were linked to the location (island). 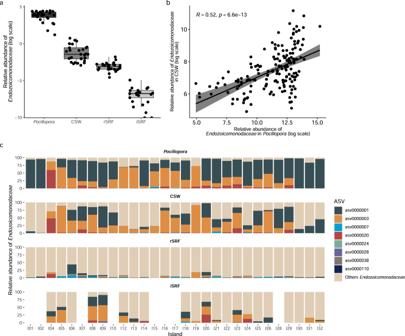Fig. 3: Relative abundance ofEndozoicomonadaceaeinPocilloporacorals and the surrounding environment. aEndozoicomonadaceaerelative abundance in the coralPocilloporahost, the colony surrounding water (CSW), the surface water over the reef (rSRF), and the surface water off the island (iSRF) in the 0.2–3 µm planktonic size fraction. The box plot horizontal bars show the median value, the box indicates the first and third QRs, and the whiskers indicate 1.5*IQR.bSpearman correlation between relative abundance ofEndozoicomonadaceaeinPocilloporaand in colony surrounding water (CSW). The lines represent the result of linear regression with the gray shadow as the 95% confidence interval. A two-sidedp-value is given.cRelative abundance of the dominantEndozoicomonadaceaeASVs in the different sampling environments at each island. Source data are provided as a Source Data file. This unique dataset from the Tara Pacific expedition reveals the taxonomic and functional diversity of coral-associated Endozoicomonadaceae and emphasizes the need for studies at the lineage level to uncover the bacterial compartment of the coral holobiont. Sample collection, environmental parameters, and biomarkers Coral and plankton samples were taken across the Pacific Ocean from three to four different sites at each of the 32 islands visited during the Tara Pacific expedition [80] . The detailed sampling protocols are presented in Lombard et al. [81] . Based on morphology, we targeted the complex Pocillopora meandrina , the robust Porites lobata and the fire coral Millepora platyphylla . Samples from 10 different colonies from each species were collected at each site using a hammer and a chisel. They were stored individually underwater in Ziploc bags, and conditioned in tubes with DNA/RNA shield (Zymo Research, Irvine, CA, USA) at −20 °C once on board. Additionally, plankton was sampled on 0.2–3 µm and 3–20 µm filters by filtering 100 L of water obtained with a pump near the islands and over the reefs, and with a diver held hose at the surface of the Pocillopora colonies. All filters were preserved in cryovials in liquid nitrogen. Because some corals within the same genus can be difficult to differentiate by eye, results are aggregated at genus level: Pocillopora , Porites and Millepora . Several environmental parameters were measured at the time of collection following the protocols detailed in Lombard et al. [81] . These include temperature and salinity measured with a CTD (Castaway CTD), nutrients quantified back in the laboratory and chlorophyll a (chla) concentrations. Sample provenance and environmental context are available on Zenodo [82] . DNA extraction and sequencing DNA was extracted with comercial kits after mecanical cell disruption. The detailled protocols for corals and plankton are presented in Belser et al. [83] . Metabarcoding sequencing targeted all 10 colonies taken at each site for each coral genus at the 32 islands. The prokaryote 16S rRNA gene was first amplified with a nested PCR approach with a first full-length amplification using the 27F/1492R 16S rRNA prokaryotic primer set [29] , [84] in order to increase the target prokaryotic DNA, and a second amplification using the 515F-Y/926R primers [85] . The Symbiodiniaceae internal transcribed spacer (ITS2) was amplified with primers SYM-VAR-5.8S2 / SYM-VAR-REV. The sequencing was performed on an Illumina sequencer to obtain 0.5 to 1 M of ~250 pb 16S rRNA paired-end reads [83] , and ~20.000 of ~250 bp paired-end reads for ITS2. Details are provided in Belser et al. [83] . Metagenomic sequencing was performed on three coral replicates from each site of a subset of 11 islands (I01-Islas de las Perlas, I02-Coïba, I03-Malpelo, I04-Rapa Nui, I05-Ducie, I06-Gambier, I07-Moorea, I08-Aitutaki, I09-Niue, I10-Upolu, and I15-Guam). The sequencing was performed on a NovaSeq6000 or HiSeq4000 Illumina sequencer (Illumina, San Diego, CA, USA) in order to produce 100 M of ~150 pb paired-end reads per sample. Details are provided in Belser et al. [83] . All sequencing files were submitted to the European Nucleotide Archive (ENA) at the EMBL European Bioinformatics Institute (EMBL-EBI) under the Tara Pacific Umbrella project PRJEB47249. Samples and their metadata were registered in the ENA biosample database. Sample provenance and environmental context are available on Zenodo [82] . 16S rRNA gene and ITS2 sequence analysis For 16S rRNA gene analysis [15] , adapters were removed with cutadapt (version 2.8) [86] and an ASV abundance table was built with DADA2 (version 1.14) [87] as detailed in the scripts published in Zenodo [88] . Samples were grouped by sequencing lane to learn errors and infer ASVs. ASVs representing less than six inserts were tagged as being spurious and removed. Taxonomic annotation was performed with IDTAXA [89] with a confidence threshold of 40 against the SILVA v.138 database. Eukaryotic ASVs (chloroplast and mitochondria) were identified based on taxonomic annotation following the criteria published in Zenodo [88] and removed from the dataset prior to analysis. In addition, bacterial sequences annotated at the family level as Oxalobacteraceae, Comamonadaceae, Cutibacterium and Yersiniaceae were identified as reagent contaminants and removed from the dataset. Symbiodiniaceae profiles were obtained using SymPortal [90] , which uses the intragenomic diversity of Symbiodiniaceae ITS2 to define ITS2 type profiles based on consistent co-occurrence of intragenomic ITS2 variants across all samples. A hierarchical clustering, using hclust function from the R “stats” package with Complete Linkage method, was performed on the unifrac matrix distance of the ITS2 abundance table to obtain Symbiodiniaceae community clusters. Host lineage assignation and phenotypic signature A set of genome-wide unlinked single nucleotide polymorphisms (SNPs), represented in >100 colonies of Pocillopora and Porites , were identified in the metagenomics dataset from the subset of 11 islands. For Millepora only target genes SNP of around 60 colonies were produced. From the analysis of these SNPs [91] we identified five independent genetic lineages in Pocillopora , three in Porites (nine geographic sub-lineages) and five in Millepora . The detailled method for host lineage assignment protocols are presented in ref. [91] . The phenotypic signatures of Pocillopora and Porites were defined through six biomarkers: the coral protein content, the Symbiodiniaceae content per coral mg of protein biomass [92] , Symbiodiniaceae content per coral surface [92] , protein ubiquitination [93] and carbonylation per coral mg of protein [94] to assess the cellular damages, and total antioxidant content per coral mg of protein to assess the cellular defenses [95] . The detailed protocols are presented in ref. [96] . 16S rRNA gene data analysis A total of 2447 metabarcoding samples of corals were analyzed. Prokaryotic and Endozoicomonadaceae community diversity were estimated by computing the Shannon index with the function diverse from “diverse” R package [97] . In order to account for the compositional characteristic of the prokaryote abundance table, data were weighted center log ratio transformed (wCLR) before computing statistics. To infer the effect of environmental factors and coral phenotypic biomarkers on Endozoicomonadaceae community composition, Kendall’s rank correlation was computed for the 32 islands using bioenv function from “vegan” R package [98] and p -value were adjusted using Benjamini et Hochberg [99] method. The correlations between Endozoicomonadaceae community composition and environmental factors, phenotypic biomarkers, coral genetic lineage, or Symbiodiniaceae assemblage were tested individually with a mantel test [100] using mantel function from “vegan” R package. The matrices were based on Euclidean distance for all datasets except for the genetic lineages that were based on RaxML [101] distances. They were computed for Pocillopora and Porites on the subset of 11 islands for which data on genetic lineages and phenotypic biomarkers were available. A variance partitioning analysis was done, using the function fitExtractVarPartModel from the “variancePartition” R package [102] , to quantify the contribution of the location (island), the coral genetic lineage, and the Symbiodiniaceae assemblage (community clusters) on Endozoicomonadaceae community composition across the subset of 11 islands. An ASVs distance tree was constructed using 16S rRNA gene sequences. Sequences were aligned with MUSCLE [103] , and the alignment was trimmed manually to remove gaps and get all sequences to start and end at the same position. A distance matrix was computed with the KIMURA model of transition and transversion rates, and the tree constructed based on the Fitch-Margoliash method, based on least squares principle, in PHYLIP [104] . Metagenomic assemblies and binning A total of 270 metagenomes (101 Pocillopora , 108 Porites and 61 Millepora ) were analyzed. Sequencing reads were quality filtered using BBMap (version 38.71) [105] by removing sequencing adapters from the reads, removing reads that mapped to quality control sequences (PhiX genome) and discarding low-quality reads using the parameters trimq = 14, maq = 20, maxns = 0 and minlength = 45. Downstream analyses were performed on quality-controlled reads, or, if specified, merged quality-controlled reads (bbmerge.sh minoverlap = 16). Quality-controlled reads were normalized (bbnorm.sh target=40, mindepth = 0) before they were assembled with metaSPAdes (version 3.12 or version 3.13 if required) [106] . The resulting scaffolded contigs (hereafter scaffolds) were finally filtered by length (≥1 kbp). The quality-controlled metagenomic reads from all samples were individually mapped against the scaffolds of each sample (270 * 270 mapping) using the Burrows-Wheeler-Algorithm (BWA)(version 0.7.17-r1188) [107] . Alignments were filtered to be at least 45 bases in length, with an identity of ≥97% and covering ≥80% of the read sequence. The resulting BAM files were processed using the jgi_summarize_bam_contig_depths script of MetaBAT2 (version 2.152.1) [108] to provide within- and between-sample coverages for each scaffold.v5. The scaffolds were finally clustered into bins for each metagenomic sample with the automatic algorithm MetaBAT2 (version 2.15) using parameters –minContig –2000 and maxEdges 500 to increase sensitivity. The quality of each metagenomic bin was evaluated using both the ‘lineage workflow’ of CheckM (version 1.1.1) [109] and Anvi’o (version 6.1) [110] . Metagenomic bins for which either CheckM/Anvi’o reported a completeness/completion ≥30% and a contamination/redundancy ≤10% were taxonomically annotated using GTDB-Tk (version 1.0.2) [111] with default parameters against the GTDB r89 release [112] in order to select Endozoicomonadaceae bacteria. The 27 identified bins are available on Zenodo ( https://zenodo.org/record/7840163 ). Species-level profiling with mOTUs and mTAGs Metagenomic bins that passed the quality filtering were additionally added to the database (version 2.5.1) of the metagenomic profiling tool mOTUs [113] to generate an extended mOTUs reference database, following the approach of Paoli et al. [114] . Only genomes with at least six out of the ten universal single-copy marker genes as identified by fetchMGs (version 1.1) [115] were used. The species-level profiling was then computed by mapping quality-controlled metagenomic reads against this extended database using default parameters of mOTUs (version 2). Taxonomic profiling using degenerate consensus reference sequences of ribosomal RNA genes was performed with mTAGs (version 1.0) [116] on metagenomic reads samples. Selection of Endozoicomonadaceae from databases All available Endozoicomonadaceae genomes (24) and closely related (two Zooshikella ) were downloaded from the NCBI genomes database (last accessed November 2021). Additionally, five Endozoicomonas genome assemblies from Neave et al. 2017 [23] were recovered from the authors and two putative Endozoicomonadaceae genomes (CAR1_bin20 and CAR3_bin23) assembled in Robbins et al. [117] reobtained from https://data.ace.uq.edu.au/public/sponge_mags . External genomes were taxonomically checked using GTDB-Tk as described for the metagenomic bins. Quality evaluations of Endozoicomonadaceae bins and genomes The quality of each Endozoicomonadaceae bins and added genomes from the literature was assessed using the ‘lineage workflow’ of CheckM (version 1.1.1) [109] and Anvi’o (version 6.1) [110] . Endozoicomonadaceae bins with a completeness ≥50% and a contamination ≤10% were kept for downstream analysis and will be referred to as Metagenome Assembled Genomes (MAGs) or genomes. The three new Endozoicomonadaceae species described in the present study ( Endozoicomonas pocilloporae , Parendozoicomonas poriteae and Endozoicomonas milleporae ) have been deposited in the SeQCode registry [118] . Genes calling and annotation Gene calling was performed using Prodigal (version 2.6.3) [119] and ribosomal RNAs were extracted using HMMER (version 3.3.2) [120] . These steps were performed with Anvi’o (version 6.1) by following the procedure described here: https://merenlab.org/2016/06/22/anvio-tutorial-v2 . The predicted proteins recovered from Endozoicomonadaceae genomes were annotated by identifying protein domain family with HMMER searches ( http://hmmer.org/ ) against the PfamA database (version 33.1) [121] and by assigning orthologous groups (OGs) using eggNOG-mapper (version 2.0.1) [122] , [123] based on eggNOG database (version 5.0) [124] . KEGG [125] and InterProscan [126] annotation was inferred from the OGs annotation. Based on this annotation, completion of metabolic modules/pathways was accessed using the information available from KEGG Metabolic pathways [125] and MetaCyc Metabolic Pathway Database [127] . Annotation of the predicted proteins was also performed using the HMMs from dbCAN (Version 11) to identify Carbohydrate-Active Enzymes (CAZy) [128] . Comparative genomic analysis The phylogenomic tree of Endozoicomonadaceae was inferred using a concatenated alignment of 71 bacterial single-copy marker proteins as detailed by the Anvi’o ( https://anvio.org/ ). The tree included MAGs from this study as well as reference genomes from earlier studies that had ≥61 single-copy markers. The tree was visualized and annotated using the iTOL (version 6.4.1) [129] . Average nucleotide identity (ANI) between Endozoicomonadaceae genomes were calculated using PyANI implemented in Anvi’o (version 6.1). Pairwise amino acid identity (AAI) between genomes was computed using comparem tool ( similarity and aai command) ( https://github.com/dparks1134/CompareM ). In order to provide a species-level clustering of genomes, dRep (version 3.1.1) [130] with a 95% ANI threshold [131] and SpecI [132] reused on all genomes. Endozoicomonadaceae MAGs within the same genome cluster were grouped into subclades based on mean ANI value ≥ 98% and host species lineage isolation source. Newly identified Endozoicomonadaceae species were named according to the host genus and subclade according to the genetic lineage of the host. Coral genomes Coral genomes assembly and annotation protocols are detailed in Noel et al. 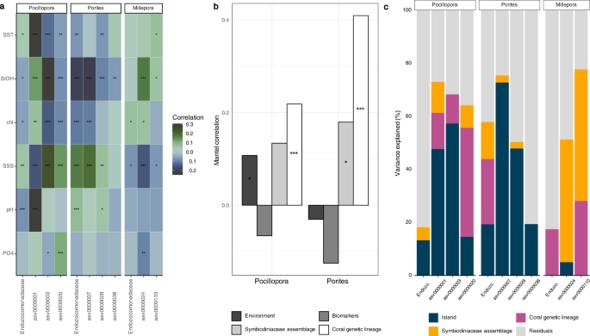Fig. 4: Correlation betweenEndozoicomonadaceae, environment, islands, host genetic lineages, Symbiodiniaceae symbionts, and phylotypic biomarkers. aKendall correlations across 32 islands between abundantEndozoicomonadaceaeASVs and environmental factors.Pocillopora(n= 889 samples),Porites(n= 903), andMillepora(n= 515). SST: Sea Surface Temperature; SiOH: Silanol; chl: Chlorophyll a; SSS: Sea Surface Salinity; pH; PO4: phosphate.bMantel correlation across 11 islands betweenEndozoicomonadaceacommunity composition and environmental conditions, phylotypic biomarkers, Symbiodiniaceae assemblages and coral host genetic lineages for the two coral generaPocillopora(n= 77) andPorites(n= 80) phylotypic biomarkers data forMilleporaare missing).cVariance partition analysis explaining the variance of the relative abundance ofEndozoicomonadaceaeand individual ASVs across 11 islands in relation to island, coral genetic lineages and Symbiodiniaceae assemblages inPocillopora(n= 96), Porites(n= 99),andMillepora(n= 55). Source data are provided as a Source Data file. [133] . Briefly, Pocillopora cf. effusa , Porites lobata colonies were collected at Moorea, French Polynesia. An amount of 15 g of each coral colony was stored at −80 °C, after flash freezing using liquid nitrogen, until DNA extraction. The genomes were sequenced using a combination of long (Oxford Nanopore Technologies, ONT) and short reads (Illumina). 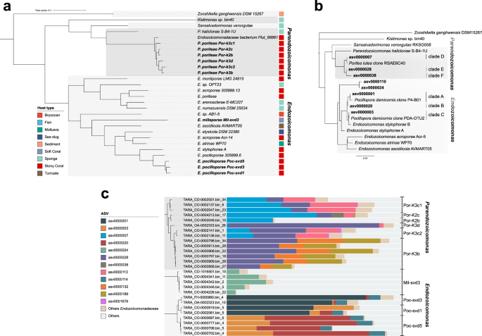Fig. 5: Distance tree of Endozoicomonadaceae. aBased on 71 concatenated single-copy marker proteins from MAGs andbbased on 16S rRNA genes from ASVs. Clades were defined in this study. ASVs and MAGs from this study are in bold.cProportion of ASVs in the samples from which the MAGs were reconstructed. 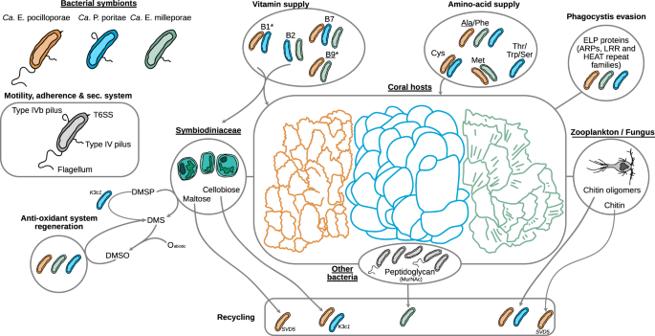Fig. 6: Schematic summary of the inferred metabolisms and appendages characterizing the three new species and lineages (SVD5, K3c1) ofEndozoicomonadaceaefound inPocillopora (orange), Porites (blue), and Millepora (green). Underlined names: vitamin or amino acid also produced by the coral host, asterisk: genes for export not known. T6SS: type 6 secretion system, ELP: eukaryotic like protein, ARPs: actin-related proteins, LRR: leucine-rich repeats, DMSP: dimethylsulfoniopropionate, DMSO: dimethylsulfoxide, DMS: Dimethyl sulfide. To generate long-reads based genome assemblies four different assemblers were used: Smartdenovo [134] , Redbean [135] , Flye [136] , and Ra [137] . From the assemblies genes calling was performed and were functionally assigned by aligning them against the nr database [138] (NCBI) using diamond [139] (version 0.9.24). Reporting summary Further information on research design is available in the Nature Portfolio Reporting Summary linked to this article.